Prostaglandin E2 and SOCS1 have a role in intestinal immune tolerance Interleukin 10 (IL-10) and regulatory T cells (Tregs) maintain tolerance to intestinal microorganisms. However, Il10 −/− Rag2 −/− mice, which lack IL-10 and Tregs, remain healthy, suggesting the existence of other mechanisms of tolerance. Here, we identify suppressor of cytokine signalling 1 (SOCS1) as an essential mediator of immune tolerance in the intestine. Socs1 −/− Rag2 −/− mice develop severe colitis, which can be prevented by the reduction of microbiota and the transfer of IL-10-sufficient Tregs. Additionally, we find an essential role for prostaglandin E2 (PGE2) in the maintenance of tolerance within the intestine in the absence of Tregs. Socs1 −/− dendritic cells are resistant to PGE2-mediated immunosuppression because of dysregulated cytokine signalling. Thus, we propose that SOCS1 and PGE2, potentially interacting together, act as an alternative intestinal tolerance mechanism distinct from IL-10 and Tregs. Several mechanisms, including immunoregulation by the innate and adaptive immune systems, allow for millions of bacteria to symbiotically reside in the gastrointestinal tract without disruption of gut homeostasis. Breakdown of tolerance to intestinal microorganisms could have a fundamental role in the pathogenesis of inflammatory bowel disease (IBD). Previous studies of several genetically engineered mouse models have shown that lack of immunosuppression leads to colitis, for example, Il2 −/− and Il10 −/− , and dominant-negative transforming growth factor-β (TGF-β) type 2 receptor transgenic (Tg) mice develop spontaneous colitis [1] . The major targets of interleukin 2 (IL-2) and TGF-β are T cells: TGF-β suppresses the growth of T cells and their differentiation into Th1 and Th2 cell subsets [2] , and both TGF-β and IL-2 are required for the induction, maintenance or function of Foxp3-expressing regulatory T cells [3] (Foxp3 + Tregs, hereafter referred to as Tregs). IL-10, on the other hand, suppresses the activation of innate immune cells in response to various Toll-like receptor stimuli through a transcription factor signal transducer and activator of transcription 3 (STAT3) [4] . The Tregs constitute a distinct population of CD4 + T cells that have an essential role in the maintenance of systemic tolerance. Alterations in Treg function lead to the activation of T-helper cell subsets known as Th1, Th2 and Th17, which produce the cytokines interferon-γ (IFNγ), IL-4 and IL-17, respectively, as well as to various types of systemic inflammation including inflammation of the gut. However, Rag1 −/− mice lacking Tregs do not develop colitis spontaneously. Furthermore, Tgfb1 −/− Rag2 −/− and Stat3 −/− Rag2 −/− mice do not develop colitis despite their lack of Tregs, TGF-β and IL-10 signalling [5] , [6] . Therefore, another tolerance mechanism, in addition to TGF-β and IL-10, must exist in the innate immune system. Many inflammatory cytokines use the janus kinase (JAK)/STAT signalling pathway, which is strictly regulated by negative regulatory mechanisms that limit excessive signalling. Two particularly important players in this negative regulation are the proteins known as suppressor of cytokine signalling 1 (SOCS1) and SOCS3. SOCS1 regulates the signals of various cytokines such as IFNγ, IL-2, IL-4, and IL-7 (ref. 7 ) Socs1 −/− mice die as early as 2 to 3 weeks after birth as result of severe inflammation in the liver [8] , though they survived much longer in the absence of IFNγ or in T-cell-deficient conditions. In this study, we show that Socs1 −/− Rag2 −/− mice develop severe spontaneous T-cell-independent colitis. Adoptive transfer of IL-10-sufficient Tregs suppressed the colitis of Socs1 −/− Rag2 −/− mice, suggesting that SOCS1 is necessary to maintain the innate immune tolerance in the intestine in the absence of Tregs. IL-10 and IL-10-sufficient Tregs suppressed the production of inflammatory cytokines from lipopolysaccharide (LPS)-stimulated bone marrow-derived dendritic cells (BMDCs), and Socs1 −/− BMDCs were as sensitive to IL-10-mediated suppression as Socs1 +/+ BMDCs were. Therefore, we hypothesized that there is another immunosuppressive mechanism in the intestinal innate immune system, whose function is impaired in Socs1 −/− cells, and we sought to identify factors required for this distinct mechanism of immune suppression. Prostaglandin E2 (PGE2) is an IL-10-independent innate immune suppressor, and SOCS1-deficiency abolished its immunosuppressive effect. Furthermore, deprivation of PGE2 by cyclooxygenase (COX) inhibitor provoked severe colitis in Rag2 −/− but not in Rag2 +/+ mice, which was also prevented by the transfer of Tregs. Thus, we propose that the tolerance in the intestinal innate immune system is regulated by a unique mechanism involving PGE2, the suppressive effect of which could be overridden by inflammatory cytokine signalling, which is strictly regulated by SOCS1. Socs1 −/− Rag2 −/− mice develop spontaneous colitis Socs1 −/− mice die shortly after birth as result of severe systemic inflammation [8] . It has been shown that early lethality can be reverted by crossing with Ifng −/− mice, Tcra −/− mice or Rag2 −/− mice, or by restoring SOCS1 expression in T and B cells by crossing with T- and B-cell-specific Socs1 Tg mice ( Socs1 -KOTg mice) [8] , [9] , [10] , [11] . 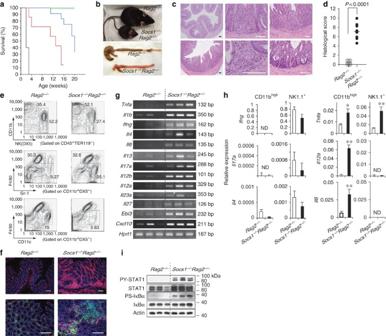Figure 1:Socs1−/−Rag2−/−mice develop spontaneous colitis. (a) The survival curves ofSocs1−/−(black,n=5),Socs1−/−Tcra−/−(red,n=14),Socs1−/−Rag2−/−(blue,n=12),Socs1-KOTg (green,n=6) andIfng−/−Socs1−/−(green, dotted,n=10) mice. (b)Rag2−/−andSocs1−/−Rag2−/−mice (8-week-old; upper panel). Representative macroscopic observations of the colons of 9-week-oldRag2−/−andSocs1−/−Rag2−/−mice (lower panel). (c) Representative histopathology of the colons ofRag2−/−(upper left panel) andSocs1−/−Rag2−/−mice (other five panels) at 9 weeks of age stained with haematoxylin and eosin. Scale bar, 100 μm. (d) The histological scores of colitis forRag2−/−(n=9) andSocs1−/−Rag2−/−(n=8) mice at 9 weeks of age. The horizontal lines indicate the mean values. (e) Flow cytometric analyses showing the proportions of CD11bhighand natural killer (NK) (DX5+) cells among CD45+TER119−cells (upper), Gr-1+and F4/80+cells among CD11b+cells (middle) and CD11c+and F4/80+cells among CD11b+cells (lower) in the spleens ofRag2−/−andSocs1−/−Rag2−/−mice. Data are representative of three independent experiments. (f) Fluorescence immunohistochemistry showing the infiltration of CD45+cells (red) into the colonic lamina propria ofRag2−/−(upper left panel) andSocs1−/−Rag2−/−mice (upper right panel). The infiltrating CD45+cells were predominantly CD11b+cells (green), although NK1.1+cells (red) were also significantly increased (lower panels). Nuclei of cells are stained with Hoechst 33342 dye (blue). Data are representative of three independent experiments using samples from different mice. Scale bar, 100 μm. (g) RNAs were extracted from the colons of 9-week-oldRag2−/−andSocs1−/−Rag2−/−mice, and the indicated gene expression was analysed by RT-PCR. Three mice per group are shown. Data are representative of three independent experiments using different samples from one to three mice per group. (h) CD11bhighNK1.1−and NK1.1+cells were sorted by FACSAria from the spleens ofRag2−/−andSocs1−/−Rag2−/−mice, and RNA was purified from the cells. The relative expression levels of the indicated genes were normalized againstHprt1using Ct values determined by quantitative real-time RT-PCR. Error bars represent +s.d. of triplicate measurements for each sample. *P<0.05 and **P<0.01 compared withRag2−/−cells. Data are representative of two independent experiments. (i) Proteins were extracted from the colons of 9-week-oldRag2−/−andSocs1−/−Rag2−/−mice, and western blot analyses were performed using indicated Abs. Three mice per group are shown. PY, tyrosine phosphorylated; PS, serine phosphorylated. Data are representative of two independent experiments using different samples from two to three mice per group. ND, not determined. Figure 1a shows the course of survival of various Socs1 −/− mice in our facility. These data suggest that dysregulation of IFNγ signalling and activation of lymphocytes are the main causes of the early lethality in Socs1 −/− mice. We have previously shown that Socs1 −/− Tcra −/− mice developed more severe colitis than Tcra −/− mice [11] . We suspected that SOCS1 deficiency in T cells might contribute to the development of colitis; however, we later found that Socs1 -KOTg mice, in which SOCS1 expression is restored in T cells, also developed mild colitis with age [12] . Furthermore, we found that Socs1 −/− Rag2 −/− mice developed fatal colitis ( Fig. 1 ). These observations suggest that SOCS1 expression in cells other than T cells is important in suppression of colitis. Figure 1: Socs1 −/− Rag2 −/− mice develop spontaneous colitis. ( a ) The survival curves of Socs1 −/− (black, n =5), Socs1 −/− Tcra −/− (red, n =14), Socs1 −/− Rag2 −/− (blue, n =12), Socs1 -KOTg (green, n =6) and Ifng −/− Socs1 −/− (green, dotted, n =10) mice. ( b ) Rag2 −/− and Socs1 −/− Rag2 −/− mice (8-week-old; upper panel). Representative macroscopic observations of the colons of 9-week-old Rag2 −/− and Socs1 −/− Rag2 −/− mice (lower panel). ( c ) Representative histopathology of the colons of Rag2 −/− (upper left panel) and Socs1 −/− Rag2 −/− mice (other five panels) at 9 weeks of age stained with haematoxylin and eosin. Scale bar, 100 μm. ( d ) The histological scores of colitis for Rag2 −/− ( n =9) and Socs1 −/− Rag2 −/− ( n =8) mice at 9 weeks of age. The horizontal lines indicate the mean values. ( e ) Flow cytometric analyses showing the proportions of CD11b high and natural killer (NK) (DX5 + ) cells among CD45 + TER119 − cells (upper), Gr-1 + and F4/80 + cells among CD11b + cells (middle) and CD11c + and F4/80 + cells among CD11b + cells (lower) in the spleens of Rag2 −/− and Socs1 −/− Rag2 −/− mice. Data are representative of three independent experiments. ( f ) Fluorescence immunohistochemistry showing the infiltration of CD45 + cells (red) into the colonic lamina propria of Rag2 −/− (upper left panel) and Socs1 −/− Rag2 −/− mice (upper right panel). The infiltrating CD45 + cells were predominantly CD11b + cells (green), although NK1.1 + cells (red) were also significantly increased (lower panels). Nuclei of cells are stained with Hoechst 33342 dye (blue). Data are representative of three independent experiments using samples from different mice. Scale bar, 100 μm. ( g ) RNAs were extracted from the colons of 9-week-old Rag2 −/− and Socs1 −/− Rag2 −/− mice, and the indicated gene expression was analysed by RT-PCR. Three mice per group are shown. Data are representative of three independent experiments using different samples from one to three mice per group. ( h ) CD11b high NK1.1 − and NK1.1 + cells were sorted by FACSAria from the spleens of Rag2 −/− and Socs1 −/− Rag2 −/− mice, and RNA was purified from the cells. The relative expression levels of the indicated genes were normalized against Hprt1 using Ct values determined by quantitative real-time RT-PCR. Error bars represent +s.d. of triplicate measurements for each sample. * P <0.05 and ** P <0.01 compared with Rag2 −/− cells. Data are representative of two independent experiments. ( i ) Proteins were extracted from the colons of 9-week-old Rag2 −/− and Socs1 −/− Rag2 −/− mice, and western blot analyses were performed using indicated Abs. Three mice per group are shown. PY, tyrosine phosphorylated; PS, serine phosphorylated. Data are representative of two independent experiments using different samples from two to three mice per group. ND, not determined. Full size image Socs1 −/− Rag2 −/− mice showed marked growth retardation, but survived for up to 4 or 5 months after birth ( Fig. 1a and b ). All Socs1 −/− Rag2 −/− mice developed severe colitis at 8–9 weeks of age, suffering from diarrhoea and weight loss, whereas littermate Rag2 −/− mice housed in the same cage never developed colitis ( Fig. 1b–d ). Through histological examination, we observed many mononuclear and polymorphonuclear cells infiltrating the lamina propria of the large intestines of Socs1 −/− Rag2 −/− mice ( Fig. 1c ). The inflammation extended from the caecum to the rectum, accompanied by the elongation of the crypts, goblet cell depletion and crypt abscesses, all of which are characteristic of chronic colitis. Flow cytometric analyses showed that CD11b high cells and natural killer cells were predominant in the spleens of both Rag2 −/− and Socs1 −/− Rag2 −/− mice ( Fig. 1e ). There was an increase in CD11b high cells and Gr-1 + cells in Socs1 −/− Rag2 −/− mice, probably reflecting granulocytosis caused by active colitis. Immunohistochemical examination showed massive infiltration of CD45 + cells in the lamina propria of Socs1 −/− Rag2 −/− mice ( Fig. 1f ). Most of these infiltrating cells were also stained with anti-CD11b or NK1.1, both of which stained significantly more cells in Socs1 −/− Rag2 −/− colons than in Rag2 −/− colons ( Fig. 1f ). mRNA levels of most of the inflammatory cytokines were upregulated in the colons of Socs1 −/− Rag2 −/− mice ( Fig. 1g ). To determine the source of these cytokines, we sorted CD11b high NK1.1 − and CD11b low NK1.1 + cells, and performed quantitative reverse transcription PCR ( Fig. 1h ). IL-12p35 and IL-6 were produced almost exclusively by the CD11b + cells, whereas tumour necrosis factor-α (TNFα) was produced by both CD11b + and NK1.1 + cells ( Fig. 1h ). The expression levels of these cytokines were upregulated in the Socs1 −/− group. IFNγ was produced only by NK1.1 + cells. NK1.1 + cells also expressed small amounts of IL-17A and IL-4. The production of IL-17 from NK1.1 + cells has also been reported by Passos et al . [13] . Although the expression levels of IFNγ, IL-4 and IL-17A were upregulated in the colons of Socs1 −/− Rag2 −/− mice ( Fig. 1g ), the expression levels of these cytokines per cell in Socs1 −/− NK1.1 + cells were similar to or less than those in Socs1 +/+ NK1.1 + cells ( Fig. 1h ). Therefore, the upregulation of these cytokines in the tissue seemed to be due to the increase in the number of infiltrating cells. Western blot analyses showed that phosphorylation of STAT1 and IκBα was significantly augmented in the colons of Socs1 −/− Rag2 −/− mice, suggesting the activation of JAK/STAT1 and nuclear factor-κB pathways in these mice ( Fig. 1i ). Characterization of the colitis of Socs1 −/− Rag2 −/− mice Socs1 −/− Rag2 −/− mice treated with broad-spectrum antibiotics from 6 weeks of age never developed colitis even at 9 weeks of age. Furthermore, colitis was markedly improved by antibiotic treatment even after it had developed ( Fig. 2a ). These observations suggest that Socs1 −/− intestinal innate immune cells were highly activated by intestinal commensal bacteria, resulting in the production of inflammatory cytokines, which leads to the development of spontaneous colitis. 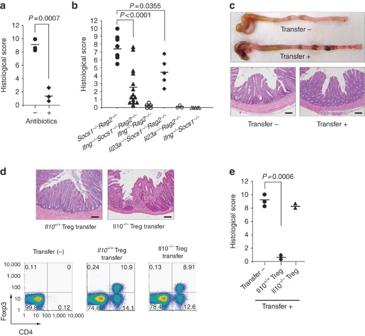Figure 2: Characterization of the colitis inSocs1−/−Rag2−/−mice. (a) Histological scores of the colitis of 16-week-oldSocs1−/−Rag2−/−mice treated with or without antibiotics for 2 weeks from 14 weeks of age (n=3). The horizontal lines indicate the mean values. (b) Histological scores of the colitis ofSocs1−/−Rag2−/−mice (black circles,n=7),Ifng−/−Socs1−/−Rag2−/−mice (black triangles,n=14),Ifng−/−Rag2−/−mice (white circles,n=5),Il23a−/−Socs1−/−Rag2−/−mice (black diamonds,n=5),Il23a−/−Rag2−/−mice (white diamonds,n=3) andIfng−/−Socs1−/−mice (white triangles,n=5) at 9 weeks of age. The horizontal lines indicate the mean values. (c) Macroscopic and microscopic observations of the colons ofSocs1−/−Rag2−/−mice with or without Treg transfer. CD4+CD25highT cells (2×105cells) sorted from WT mice were transferred at 10 weeks of age. The mice were killed 6 weeks after the transfer. Representative data are shown. Scale bar, 200 μm. (d) Representative histopathology of the colons ofSocs1−/−Rag2−/−mice transferred with Tregs sorted from WT (Il10+/+) andIl10−/−mice. Scale bar, 100 μm (upper panel). The reconstitution of Tregs confirmed by flow cytometry (lower panel). Spleens were removed fromSocs1−/−Rag2−/−mice without Treg transfer (lower left) or 6 weeks after the transfer with the indicated Tregs (lower middle and right), and the frequencies of CD4+and Foxp3+cells among TER119−CD11c−cells gated on particular forward and side scatter were analysed. At 6 weeks after the transfer, nearly 40% of the CD4+cells expressed Foxp3, and the frequency was similar between theIl10+/+andIl10−/−Treg-transferred group. (e) Histological scores of the colitis of 16-week-oldSocs1−/−Rag2−/−mice without transfer (black circles,n=3), transferred withIl10+/+Tregs (black diamonds,n=3) and transferred withIl10−/−Tregs (black triangles,n=2) is shown. The horizontal lines indicate the mean values. Figure 2: Characterization of the colitis in Socs1 −/− Rag2 −/− mice. ( a ) Histological scores of the colitis of 16-week-old Socs1 −/− Rag2 −/− mice treated with or without antibiotics for 2 weeks from 14 weeks of age ( n =3). The horizontal lines indicate the mean values. ( b ) Histological scores of the colitis of Socs1 −/− Rag2 −/− mice (black circles, n =7), Ifng −/− Socs1 −/− Rag2 −/− mice (black triangles, n =14), Ifng −/− Rag2 −/− mice (white circles, n =5), Il23a −/− Socs1 −/− Rag2 −/− mice (black diamonds, n =5), Il23a −/− Rag2 −/− mice (white diamonds, n =3) and Ifng −/− Socs1 −/− mice (white triangles, n =5) at 9 weeks of age. The horizontal lines indicate the mean values. ( c ) Macroscopic and microscopic observations of the colons of Socs1 −/− Rag2 −/− mice with or without Treg transfer. CD4 + CD25 high T cells (2×10 5 cells) sorted from WT mice were transferred at 10 weeks of age. The mice were killed 6 weeks after the transfer. Representative data are shown. Scale bar, 200 μm. ( d ) Representative histopathology of the colons of Socs1 −/− Rag2 −/− mice transferred with Tregs sorted from WT ( Il10 +/+ ) and Il10 −/− mice. Scale bar, 100 μm (upper panel). The reconstitution of Tregs confirmed by flow cytometry (lower panel). Spleens were removed from Socs1 −/− Rag2 −/− mice without Treg transfer (lower left) or 6 weeks after the transfer with the indicated Tregs (lower middle and right), and the frequencies of CD4 + and Foxp3 + cells among TER119 − CD11c − cells gated on particular forward and side scatter were analysed. At 6 weeks after the transfer, nearly 40% of the CD4 + cells expressed Foxp3, and the frequency was similar between the Il10 +/+ and Il10 −/− Treg-transferred group. ( e ) Histological scores of the colitis of 16-week-old Socs1 −/− Rag2 −/− mice without transfer (black circles, n =3), transferred with Il10 +/+ Tregs (black diamonds, n =3) and transferred with Il10 −/− Tregs (black triangles, n =2) is shown. The horizontal lines indicate the mean values. Full size image Because SOCS1 is a strong negative regulator of the IFNγ signal, we generated Ifng −/− Socs1 −/− Rag2 −/− mice to examine the contribution of IFNγ to this colitis. As expected, Ifng deficiency significantly reduced the severity of colitis induced by Socs1 / Rag2 deficiency ( Fig. 2b ). However, Ifng deficiency did not eliminate colitis completely, suggesting that other cytokines that are highly activated in Socs1 −/− Rag2 −/− mice are also involved in colitis. An obvious candidate was IL-23. IL-23 is regarded as a key inflammatory factor involved in the pathogenesis of colitis [14] . The involvement of IL-23 in the aggravation of colitis in T-cell-deficient mice has also been reported by previous studies [15] , [16] , and the mRNA level of Il23a was increased in the colons of Socs1 −/− Rag2 −/− mice ( Fig. 1g ). To test the possibility that IL23 was involved in colitis, we generated Il23a −/− Socs1 −/− Rag2 −/− mice. Milder colitis was observed in the Il23a −/− Socs1 −/− Rag2 −/− mice than in the Socs1 −/− Rag2 −/− mice ( Fig. 2b ), which supports the idea that not only IFNγ but also IL-23 is involved in the T-cell-independent development of colitis. Interestingly, Ifng −/− Socs1 −/− mice never developed colitis, whereas Ifng −/− Socs1 −/− Rag2 −/− mice did ( Fig. 2b ). This suggests that the development of colitis caused by SOCS1 deficiency was because of the lack of functional T and B cells. These observations strongly suggest that lymphocytes have a protective role in the suppression of colitis caused by SOCS1 deficiency. Among the lymphocytes, Tregs are the most likely to be involved in this process. To explore this possibility, we transferred CD4 + CD25 high cells from wild-type (WT) mice to Socs1 −/− Rag2 −/− mice. As we expected, there was a marked reduction in the severity of colitis in the Treg-transferred group ( Fig. 2c ). In contrast, when we transferred IL-10-deficient Tregs, there was no significant improvement, despite the similarity of reconstitution rates ( Fig. 2d and e ). On the basis of these observations, we concluded that the lack of Treg-derived IL-10 is an important component in the development of colitis in Socs1 −/− Rag2 −/− mice. PGE2 as an immunosuppressor molecule in the colonic mucosa Our Treg transfer experiment into Socs1 −/− Rag2 −/− mice indicated that suppression by Treg-derived IL-10 could overwhelm the inflammatory effect of SOCS1 deficiency. In accordance with this scenario, IL-10 suppressed the TNFα and IL-12p70 production from Socs1 −/− BMDCs stimulated with LPS or LPS+IFNγ as efficiently as from Socs1 +/+ BMDCs ( Fig. 3a , data for LPS alone shown in Supplementary Fig. S1a ). Similarly, Tregs suppressed inflammatory cytokine production from BMDCs in an IL-10-dependent manner and this Treg-mediated suppression was also observed in Socs1 −/− BMDCs ( Fig. 3b ). These observations suggested that IL-10/Treg-mediated suppression was not impaired by SOCS1 deficiency; therefore, we hypothesized that another immunosuppressive mechanism was altered in the colons of Socs1 −/− Rag2 −/− mice. 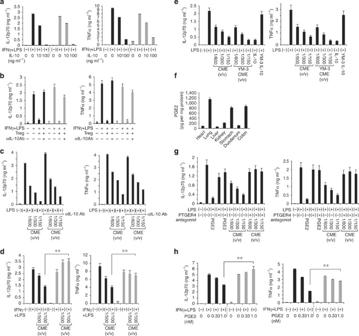Figure 3: IFNγ rendersSocs1−/−BMDCs resistant to PGE2 but not to IL-10. (a–e,g,h)Socs1+/+(black bars) andSocs1−/−(grey bars) BMDCs (5×105cells per ml) induced from the bone marrow cells ofRag2−/−andSocs1−/−Rag2−/−mice were stimulated for 12 h with indicated reagents, and the levels of IL-12p70 and TNFα in the culture supernatant were measured by ELISA. Error bars represent +s.d. Cells were stimulated in triplicate wells for each condition and s.d. was calculated from the values determined by ELISA. (a)Socs1+/+andSocs1−/−BMDCs were stimulated with LPS (10 ng ml−1) and murine IFNγ (10 ng ml−1) in the presence of graded concentrations of recombinant murine IL-10. (b)Socs1+/+andSocs1−/−BMDCs were co-cultured with 2.5×105cells per ml of CD4+CD25highT cells in the presence of soluble anti-CD3 Ab (1 μg ml−1). Cells were stimulated with LPS+IFNγ (10 ng ml−1each) with or without anti-IL-10-neutralizing Ab (αIL-10 Ab, 10 μg ml−1). (c)Socs1+/+BMDCs were stimualted with LPS (10 ng ml−1) in the presence or absence of graded concentrations of CME and αIL-10 Ab (10 μg ml−1). (d)Socs1+/+andSocs1−/−BMDCs were stimulated with LPS+IFNγ (10 ng ml−1each) in the presence of graded concentrations of CME (v/v, volume of CME/volume of solution (media+CME)). **P<0.01. (e)Socs1+/+BMDCs were stimulated with LPS (10 ng ml−1) in the presence or absence of graded concentrations of CME. The CME filtrated through YM-3 ultrafiltration columns (Millipore), which remove molecules higher than 3,000 Da, retained a suppressive function. IL-10 was used as an experimental control. (f) Tissue extracts from the indicated organs were prepared as described in the Methods, and the levels of PGE2 were determined by ELISA. Error bars indicate +s.d. of triplicate ELISA measurements for each sample. (g)Socs1+/+BMDCs were stimulated with LPS (10 ng ml−1) in the presence of PGE2 (1 nM) or graded concentrations of CME with or without PTGER4 antagonist (ONO-AE3-208; 100 nM). (h)Socs1+/+andSocs1−/−BMDCs were stimulated with LPS+IFNγ (10 ng ml−1each) in the presence of graded concentrations of PGE2. **P<0.01. Data are representative of two (f) to three (a–e,g,h) independent experiments. Figure 3: IFNγ renders Socs1 −/− BMDCs resistant to PGE2 but not to IL-10. ( a – e , g , h ) Socs1 +/+ (black bars) and Socs1 −/− (grey bars) BMDCs (5×10 5 cells per ml) induced from the bone marrow cells of Rag2 −/− and Socs1 −/− Rag2 −/− mice were stimulated for 12 h with indicated reagents, and the levels of IL-12p70 and TNFα in the culture supernatant were measured by ELISA. Error bars represent +s.d. Cells were stimulated in triplicate wells for each condition and s.d. was calculated from the values determined by ELISA. ( a ) Socs1 +/+ and Socs1 −/− BMDCs were stimulated with LPS (10 ng ml −1 ) and murine IFNγ (10 ng ml −1 ) in the presence of graded concentrations of recombinant murine IL-10. ( b ) Socs1 +/+ and Socs1 −/− BMDCs were co-cultured with 2.5×10 5 cells per ml of CD4 + CD25 high T cells in the presence of soluble anti-CD3 Ab (1 μg ml −1 ). Cells were stimulated with LPS+IFNγ (10 ng ml −1 each) with or without anti-IL-10-neutralizing Ab (αIL-10 Ab, 10 μg ml −1 ). ( c ) Socs1 +/+ BMDCs were stimualted with LPS (10 ng ml −1 ) in the presence or absence of graded concentrations of CME and αIL-10 Ab (10 μg ml −1 ). ( d ) Socs1 +/+ and Socs1 −/− BMDCs were stimulated with LPS+IFNγ (10 ng ml −1 each) in the presence of graded concentrations of CME (v/v, volume of CME/volume of solution (media+CME)). ** P <0.01. ( e ) Socs1 +/+ BMDCs were stimulated with LPS (10 ng ml −1 ) in the presence or absence of graded concentrations of CME. The CME filtrated through YM-3 ultrafiltration columns (Millipore), which remove molecules higher than 3,000 Da, retained a suppressive function. IL-10 was used as an experimental control. ( f ) Tissue extracts from the indicated organs were prepared as described in the Methods, and the levels of PGE2 were determined by ELISA. Error bars indicate +s.d. of triplicate ELISA measurements for each sample. ( g ) Socs1 +/+ BMDCs were stimulated with LPS (10 ng ml −1 ) in the presence of PGE2 (1 nM) or graded concentrations of CME with or without PTGER4 antagonist (ONO-AE3-208; 100 nM). ( h ) Socs1 +/+ and Socs1 −/− BMDCs were stimulated with LPS+IFNγ (10 ng ml −1 each) in the presence of graded concentrations of PGE2. ** P <0.01. Data are representative of two ( f ) to three ( a – e , g , h ) independent experiments. Full size image To define this non-IL-10 tolerance mechanism in the intestine and to specifically identify a soluble factor that could suppress the immune response, we prepared a whole colonic mucosal extract (CME) from the colonic mucosal layer of WT mice and included this CME in the culture media for BMDCs. Interestingly, CME suppressed LPS-induced production of IL-12p70 and TNFα from BMDCs in a dose-dependent manner ( Fig. 3c ). Because this suppression was not counteracted by anti-IL-10-neutralizing antibody (Ab), IL-10 could not be involved in the suppression ( Fig. 3c ). Importantly, the suppressive effect of CME was diminished in Socs1 −/− BMDCs but not in Socs1 +/+ BMDCs when cells were stimulated with LPS+IFNγ ( Fig. 3d , data for LPS alone shown in Supplementary Fig. S1b ). In attempting to identify the factor in CME, we noticed that the suppressive factor present in CME was heat resistant ( Supplementary Fig. S1c ), and its molecular weight was estimated to be <3,000 Da by ultrafiltration ( Fig. 3e ). Thus, it seemed likely to be a small molecule rather than a protein. We had previously purified a similar factor from mouse embryonic fibroblast culture media and identified it as PGE2 (ref. 13 ). Therefore, we suspected that the factor in CME was PGE2; in agreement with this hypothesis, the CME contained a large amount of PGE2 ( ∼ 200 ng ml −1 , as determined by enzyme-linked immunosorbent assay (ELISA)). As shown in Figure 3f , extracts from the colon, lung and stomach contained substantial amounts of PGE2, suggesting that these organs have a capacity to produce a relatively large amount of PGE2 compared with other organs under physiological conditions. The suppressive effect of CME as well as PGE2 was completely counteracted by the antagonist of PGE2 receptor 4 (PTGER4, EP4 subtype), a major immunoregulatory receptor for PGE2 (ref. 17 ) ( Fig. 3g ). These data suggested that PGE2 is a major suppressor for proinflammatory cytokine production in the intestine, although additional mechanisms of tolerance may also exist. Importantly, just like that of CME, the suppressive effect of PGE2 was diminished in Socs1 −/− BMDCs when the cells were stimulated with LPS+IFNγ ( Fig. 3h ). These data indicate that the PGE2-mediated immunosuppressive mechanism was impaired in Socs1 −/− cells. PGE2 have an indispensable role in the absence of Tregs Next, to confirm that PGE2 has a regulatory role in the intestine in the absence of Tregs, we continuously administered the non-selective COX inhibitor indomethacin to WT ( Rag2 +/+ ) and Rag2 −/− mice in the drinking water. This treatment effectively suppressed the production of PGE2 in the colons of mice of both genotypes ( Fig. 4a ). Interestingly, although indomethacin-administered WT mice rarely developed symptoms, Rag2 −/− mice showed a high susceptibility to indomethacin, and developed diarrhoea and weight loss because of severe inflammation in the caecum and colon ( Fig. 4b ) accompanied by elevated levels of inflammatory cytokines ( Fig. 4c ), whereas WT mice developed almost no inflammatory changes in the intestine. When a PTGER4 agonist was administered together with indomethacin, Rag2 −/− mice did not develop colitis and wasting disease ( Fig. 4d ), suggesting that the decrease in PGE2/PTGER4 signalling is the direct cause of indomethacin-induced inflammation in Rag2 −/− mice. 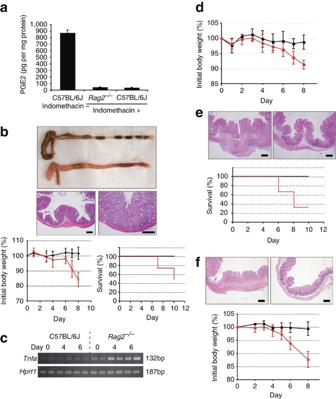Figure 4: PGE2-mediated immunosuppression is indispensable forRag2−/−but not for WT mice to avoid intestinal inflammation. (a) Mice (WT (C57BL/6J) andRag2−/−) were fed with or without 40 μg ml−1of indomethacin in drinking water for 3 days. The levels of PGE2 were determined by ELISA. (b) WT (C57BL/6J) andRag2−/−mice were continuously administered 40 μg ml−1of indomethacin in drinking water.Upper panels: Representative macroscopic and microscopic observations of the large intestines of the indomethacin-administered WT (upper intestine in macroscopic image and lower left section in microscopic image) andRag2−/−mice (lower intestine in macroscopic image and lower right section in microscopic image). Scale bar, 200 μm.Lower panels: The body weights (lower left) and survival rates (lower right) of WT (black line) andRag2−/−mice (red line) are shown;n=4 for each group. Error bars represent ±s.d. (c) RNAs were extracted from the proximal colons of the indomethacin-administered WT (C57BL/6J) andRag2−/−mice on days 0, 4 and 6 (n=2 for each day), and the indicated gene expression was analysed by RT-PCR. (d) The body weights ofRag2−/−mice administered with indomethacin alone (red line) and indomethacin plus PTGER4 agonist (black line);n=3 for each group. Error bars represent ±s.d. (e) Microscopic observations of the caecum and survival rates of indomethacin-administeredRag2−/−mice treated with antibiotics (upper right image and black line in lower panel) or without antibiotics (upper left image and red line in lower panel). Scale bar, 200 μm;n=3 for each group. (f) CD4+CD25highcells (Tregs, 2×105cells) were transferred to 4-week-oldRag2−/−mice. At 4 weeks after the transfer, mice were fed with indomethacin for 8 days. Microscopic observations of proximal colons and body weights of indomethacin-administeredRag2−/−mice transferred with Tregs (upper right image and black line in lower panel) or without Tregs (upper left image and red line in lower panel) are shown;n=3 for each group. Scale bar, 200 μm. Error bars represent ±s.d. Figure 4: PGE2-mediated immunosuppression is indispensable for Rag2 −/− but not for WT mice to avoid intestinal inflammation. ( a ) Mice (WT (C57BL/6J) and Rag2 −/− ) were fed with or without 40 μg ml −1 of indomethacin in drinking water for 3 days. The levels of PGE2 were determined by ELISA. ( b ) WT (C57BL/6J) and Rag2 −/− mice were continuously administered 40 μg ml −1 of indomethacin in drinking water. Upper panels : Representative macroscopic and microscopic observations of the large intestines of the indomethacin-administered WT (upper intestine in macroscopic image and lower left section in microscopic image) and Rag2 −/− mice (lower intestine in macroscopic image and lower right section in microscopic image). Scale bar, 200 μm. Lower panels : The body weights (lower left) and survival rates (lower right) of WT (black line) and Rag2 −/− mice (red line) are shown; n =4 for each group. Error bars represent ±s.d. ( c ) RNAs were extracted from the proximal colons of the indomethacin-administered WT (C57BL/6J) and Rag2 −/− mice on days 0, 4 and 6 ( n =2 for each day), and the indicated gene expression was analysed by RT-PCR. ( d ) The body weights of Rag2 −/− mice administered with indomethacin alone (red line) and indomethacin plus PTGER4 agonist (black line); n =3 for each group. Error bars represent ±s.d. ( e ) Microscopic observations of the caecum and survival rates of indomethacin-administered Rag2 −/− mice treated with antibiotics (upper right image and black line in lower panel) or without antibiotics (upper left image and red line in lower panel). Scale bar, 200 μm; n =3 for each group. ( f ) CD4 + CD25 high cells (Tregs, 2×10 5 cells) were transferred to 4-week-old Rag2 −/− mice. At 4 weeks after the transfer, mice were fed with indomethacin for 8 days. Microscopic observations of proximal colons and body weights of indomethacin-administered Rag2 −/− mice transferred with Tregs (upper right image and black line in lower panel) or without Tregs (upper left image and red line in lower panel) are shown; n =3 for each group. Scale bar, 200 μm. Error bars represent ±s.d. Full size image When commensal bacteria were removed by antibiotics, indomethacin did not induce colitis in Rag2 −/− mice ( Fig. 4e ), suggesting that a dysregulated immune response to commensal bacteria is involved in this colitis. Furthermore, the transfer of Tregs into Rag2 −/− mice also prevented colitis of indomethacin-treated Rag2 −/− mice ( Fig. 4f ). These findings suggest that PGE2-mediated immunosuppression is indispensable for preventing the hyperactivation of innate immune cells and the resultant intestinal inflammation under Treg-deficient conditions. Interestingly, these features of the colitis of indomethacin-treated Rag2 −/− mice were almost identical to those of the colitis observed in Socs1 −/− Rag2 −/− mice. This was consistent with our in vitro observation that the PGE2-mediated immunosuppression was impaired in Socs1 −/− BMDCs. SOCS1 maintains the immunosuppressive effect of PGE2 We attempted to ascertain how the PGE2-mediated immunosuppression was impaired in Socs1 −/− BMDCs. As mentioned in Figure 3h , the suppressive effect of PGE2 on LPS+IFNγ-induced IL-12p70 and TNFα production from BMDCs was counteracted by SOCS1 deficiency, and this antagonism was barely seen in the absence of IFNγ, suggesting that dysregulated IFNγ signal is the cause of the antagonism. When PGE2 binds to a receptor, especially PTGER4, adenylate cyclase is activated and the level of cyclic AMP (cAMP) is elevated. cAMP then suppresses the production of inflammatory cytokines by several mechanisms [18] , [19] . 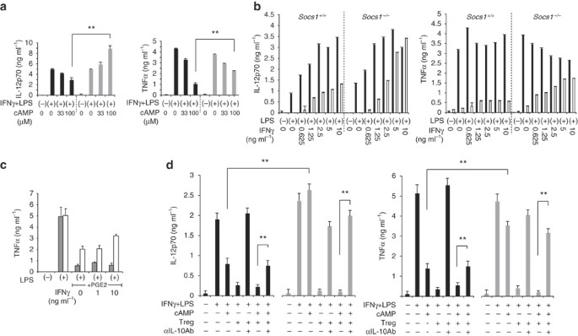Figure 5: IFNγ antagonizes cAMP but not Treg-derived IL-10 inSocs1−/−BMDCs. (a)Socs1+/+(5×105cells per ml; black bars) andSocs1−/−BMDCs (5×105cells per ml; grey bars) were stimulated with LPS+IFNγ (10 ng ml−1each) for 12 h in the presence or absence of graded concentrations of membrane-permeable cAMP analogue, 8-Br-cAMP. The levels of IL-12p70 and TNFα in the culture supernatant were measured by ELISA. (b)Socs1+/+(5×105cells per ml; left half of each panel) andSocs1−/−BMDCs (5×105cells per ml; right half of each panel) were stimulated with LPS (10 ng ml−1) for 12 h with (white bars) or without (black bars) 100 μM of 8-Br-cAMP with graded concentrations of murine recombinant IFNγ. The levels of IL-12p70 and TNFα in the culture supernatant were measured by ELISA. IFNγ dose-dependently antagonized cAMP-mediated immunosuppression, which was enhanced by SOCS1 deficiency. (c)Stat1+/+(5×105cells per ml; white bars) andStat1−/−(5×105cells per ml; grey bars) BMDCs were stimulated with LPS (10 ng ml−1) for 24 h in the absence or presence of PGE2 and graded concentrations of murine recombinant IFNγ. The level of TNFα in the culture supernatant was measured by ELISA. (d)Socs1+/+andSocs1−/−BMDCs (5×105cells per ml) were co-cultured with 2.5×105cells per ml of CD4+CD25highregulatory T cells in the presence of soluble anti-CD3 Ab (1 μg ml−1). Cells were stimulated with 10 ng ml−1of LPS+IFNγ (10 ng ml−1, each) for 12 h with or without anti-IL-10 neutralizing Ab (10 μg ml−1) in the presence or absence of membrane-permeable cAMP. The levels of IL-12p70 and TNFα in the culture supernatant were measured by ELISA. Data are representative of two (b–d) to three (a) independent experiments. Error bars represent +s.d. Cells were stimulated in triplicate wells for each condition and s.d. was calculated from the values determined by ELISA. **P<0.01. As shown in Figure 5a , Socs1 −/− BMDCs were also resistant to cAMP-mediated suppression of cytokine production in the presence of LPS+IFNγ. IFNγ dose-dependently counteracted the suppressive effects of cAMP in Socs1 −/− BMDCs ( Fig. 5b ). It is notable that IFNγ partially antagonized the suppressive effect of PGE2 and cAMP in Socs1 +/+ BMDCs ( Fig. 5b ), although this antagonism was not observed in Stat1 −/− BMDCs ( Fig. 5c ). These data suggest that the antagonistic effect of IFNγ/STAT1 pathway against PGE2 and cAMP was amplified in Socs1 −/− BMDCs. Figure 5: IFNγ antagonizes cAMP but not Treg-derived IL-10 in Socs1 −/− BMDCs. ( a ) Socs1 +/+ (5×10 5 cells per ml; black bars) and Socs1 −/− BMDCs (5×10 5 cells per ml; grey bars) were stimulated with LPS+IFNγ (10 ng ml −1 each) for 12 h in the presence or absence of graded concentrations of membrane-permeable cAMP analogue, 8-Br-cAMP. The levels of IL-12p70 and TNFα in the culture supernatant were measured by ELISA. ( b ) Socs1 +/+ (5×10 5 cells per ml; left half of each panel) and Socs1 −/− BMDCs (5×10 5 cells per ml; right half of each panel) were stimulated with LPS (10 ng ml −1 ) for 12 h with (white bars) or without (black bars) 100 μM of 8-Br-cAMP with graded concentrations of murine recombinant IFNγ. The levels of IL-12p70 and TNFα in the culture supernatant were measured by ELISA. IFNγ dose-dependently antagonized cAMP-mediated immunosuppression, which was enhanced by SOCS1 deficiency. ( c ) Stat1 +/+ (5×10 5 cells per ml; white bars) and Stat1 −/− (5×10 5 cells per ml; grey bars) BMDCs were stimulated with LPS (10 ng ml −1 ) for 24 h in the absence or presence of PGE2 and graded concentrations of murine recombinant IFNγ. The level of TNFα in the culture supernatant was measured by ELISA. ( d ) Socs1 +/+ and Socs1 −/− BMDCs (5×10 5 cells per ml) were co-cultured with 2.5×10 5 cells per ml of CD4 + CD25 high regulatory T cells in the presence of soluble anti-CD3 Ab (1 μg ml −1 ). Cells were stimulated with 10 ng ml −1 of LPS+IFNγ (10 ng ml −1 , each) for 12 h with or without anti-IL-10 neutralizing Ab (10 μg ml −1 ) in the presence or absence of membrane-permeable cAMP. The levels of IL-12p70 and TNFα in the culture supernatant were measured by ELISA. Data are representative of two ( b – d ) to three ( a ) independent experiments. Error bars represent +s.d. Cells were stimulated in triplicate wells for each condition and s.d. was calculated from the values determined by ELISA. ** P <0.01. Full size image Lastly, we confirmed the relationship among SOCS1, cAMP and IL-10/Tregs ( Fig. 5d ). When we co-cultured Socs1 +/+ BMDCs with cAMP and Tregs, the production of IL-12p70 and TNFα was intensively suppressed. The suppressive effect of Treg was diminished by anti-IL-10 Ab, indicating that Treg functioned through IL-10 in this co-culture experiment ( Fig. 5d ). Although immunosuppressive effect of cAMP was diminished in Socs1 −/− BMDCs, Tregs potently suppressed cytokine production from Socs1 −/− BMDCs in an IL-10-dependent manner ( Fig. 5d ). These phenomena were consistent with our in vivo observation that Tregs suppressed colitis in both Socs1 −/− Rag2 −/− mice and indomethacin-treated Rag2 −/− mice. We found that another STAT1-activating cytokine IL-27 and the STAT6-activating cytokines, IL-4 and IL-13, also counteracted the immunosuppressive effect of cAMP in Socs1 −/− BMDCs, although their effect was not as evident as that of IFNγ ( Fig. 6 ). This may explain why IFNγ deficiency could not completely eliminate the colitis in Ifng −/− Socs1 −/− Rag2 −/− mice ( Fig. 2b ). The involvement of STAT6-activating cytokines, especially IL-13, for pathogenesis of colitis has been shown in previous studies [20] , [21] . Although a recent study suggested a role of IL-13 for attenuation of production of IFNγ and IL-17, and the resultant colitis due to IL-10 deficiency [22] , our study here suggests a synergistic involvement of IFNγ, IL-4 and IL-13 for aggravation of colitis. Collectively, the Treg/IL-10 system seems to be more stable than the PGE2/cAMP system, as the former system was not affected by the strong cytokine signalling, especially IFNγ/STAT1 signalling, resulting from SOCS1 deficiency. The hierarchy among these suppression systems suggested by this study is shown in Figure 7 . 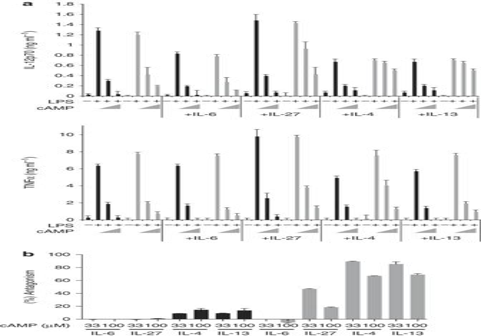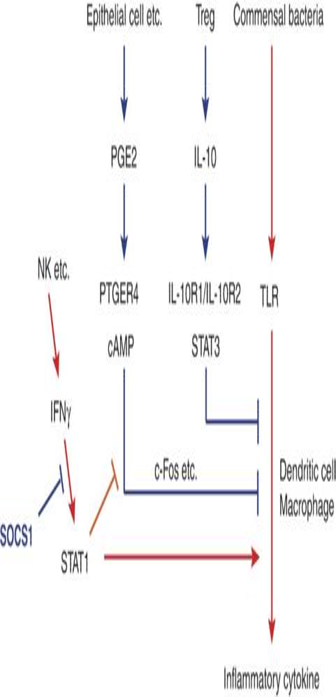Figure 7: A model for SOCS1-dependent and -independent mechanism of intestinal tolerance. Tolerance to commensal bacteria is regulated by two independent pathways: PGE2-cAMP and Treg-IL-10. Inflammatory cytokines, especially IFNγ, antagonize PGE2-cAMP-mediated suppression for Toll-like receptor signalling. SOCS1 negatively regulates IFNγ signalling, thus maintaining the PGE2-cAMP-mediated tolerance. Figure 6: Select cytokines partially antagonize the cAMP-mediated immunosuppression. Socs1+/+(5×105cells per ml; black bars) andSocs1−/−(5×105cells per ml; grey bars) BMDCs were stimulated with LPS (10 ng ml−1) and graded concentrations of 8-Br-cAMP (0, 33 and 100 mM) for 12 h with or without recombinant murine IL-6 (20 ng ml−1), IL-27 (100 ng ml−1), IL-4 (20 ng ml−1) and IL-13 (20 ng ml−1). (a) The levels of IL-12p70 and TNFα in the culture supernatant were measured by ELISA. Error bars indicate +s.d. Cells were stimulated in triplicate wells for each condition and s.d. was calculated from the values determined by ELISA. (b) The normalized antagonistic effect (% antagonism) of the indicated cytokines against the suppressive effect of cAMP for the production of IL-12p70. Data were calculated from a data set shown in panela. Data are representative of two independent experiments (a, b). Figure 6: Select cytokines partially antagonize the cAMP-mediated immunosuppression. Socs1 +/+ (5×10 5 cells per ml; black bars) and Socs1 −/− (5×10 5 cells per ml; grey bars) BMDCs were stimulated with LPS (10 ng ml −1 ) and graded concentrations of 8-Br-cAMP (0, 33 and 100 mM) for 12 h with or without recombinant murine IL-6 (20 ng ml −1 ), IL-27 (100 ng ml −1 ), IL-4 (20 ng ml −1 ) and IL-13 (20 ng ml −1 ). ( a ) The levels of IL-12p70 and TNFα in the culture supernatant were measured by ELISA. Error bars indicate +s.d. Cells were stimulated in triplicate wells for each condition and s.d. was calculated from the values determined by ELISA. ( b ) The normalized antagonistic effect (% antagonism) of the indicated cytokines against the suppressive effect of cAMP for the production of IL-12p70. Data were calculated from a data set shown in panel a . Data are representative of two independent experiments ( a, b ). Full size image Figure 7: A model for SOCS1-dependent and -independent mechanism of intestinal tolerance. Tolerance to commensal bacteria is regulated by two independent pathways: PGE2-cAMP and Treg-IL-10. Inflammatory cytokines, especially IFNγ, antagonize PGE2-cAMP-mediated suppression for Toll-like receptor signalling. SOCS1 negatively regulates IFNγ signalling, thus maintaining the PGE2-cAMP-mediated tolerance. Full size image In this study, we tried to clarify the relationship among Tregs, IL-10, PGE2 and SOCS1 in maintaining the tolerance to commensal microorganisms. Together with a previous report by Berg et al . [23] , which showed severe indomethacin-induced colitis in Il10 −/− mice, our study demonstrated the independent contributions of Treg-derived IL-10 and the PGE2/cAMP system for the maintenance of intestinal tolerance. These two systems are regarded as safeguarding each other, thus limiting the aggravation of colitis ( Fig. 7 ). Our study also suggests that inflammatory cytokine signalling would block the immunosuppressive effect of PGE2 and cAMP but not IL-10, and the absence of SOCS1 amplifies the antagonism to PGE2/cAMP. Although we have shown ex vivo that cytokine signalling regulation by SOCS1 is required for efficient PGE2-mediated suppression of activation of innate immune cells, the contribution of the resistance to PGE2/cAMP-mediated suppression in Socs1 −/− cells to the development of colitis of Socs1 −/− Rag2 −/− mice is still not clear. Because the molecular mechanisms of PGE2/cAMP-mediated innate immune suppression and STAT-dependent interference to the suppression were not fully resolved, and because we did not have a good molecular target, it was difficult for us to rescue Socs1 −/− Rag2 −/− mice from colitis by enhancing the effect of PGE2/cAMP in a manner that could avoid the effect of enhanced STATs signalling. Treatment with a PTGER4 agonist was not suitable for this purpose, because activated STATs would block the effect of the PTGER4 agonist in Socs1 −/− Rag2 −/− mice. Therefore, we could not provide direct evidence for the link between the two pathways in vivo . Nevertheless, the findings that SOCS1 and PGE2/cAMP system are indispensable for innate immune system to maintain the homeostasis in the colon in the absence of Tregs are interesting. The PGE2/cAMP system has not been well recognized as an important tolerance mechanism in vivo probably because this system is vulnerable because of the antagonism by inflammatory cytokines including IFNγ and is also masked by a strong suppressive effect of IL-10. A pivotal role of the PGE2 suppression system appeared only when Tregs or IL-10 are absent. It is well known that the administration of COX inhibitors to human IBD patients may increase the risk of relapse and worsening of the disease [20] . Similarly, the administration of a COX inhibitor has been shown to exacerbate the course of dextran sulphate sodium salt-induced colitis [21] . The IL-10/Treg system may not be fully functional in these situations. Although many mechanisms seem to be involved in the gastroprotective effect of PGE2 (ref. 24 ), suppression of the production of inflammatory cytokines is probably one of the important mechanisms for protection against colitis. The immunosuppressive activity of PGE2 largely depends on the production of cAMP from ATP. Activation of the PGE2 receptors PTGER2 (EP2) and PTGER4 (EP4) usually upregulates intracellular cAMP level, whereas PTGER1 (EP1) upregulates intracellular Ca 2+ and PTGER3 (EP3) downregulates cAMP [17] ; the anti-inflammatory effect of PGE2 is, therefore, context dependent. As shown previously, cAMP suppresses the production of inflammatory cytokines from macrophages and dendritic cells in an IL-10-independent manner [13] , [19] . Moreover, cAMP has been shown to be involved in the induction and function of Foxp3 + Tregs [25] , [26] , [27] . A recent study has shown that cAMP enhances the induction of human Th17 cells by PGE2/PTGER2/PTGER4 signalling [28] . Therefore, the effects of PGE2 and cAMP may be complicated in the presence of T cells. Nevertheless, our study established an essential role of the PGE2/cAMP system to maintain tolerance to commensal bacteria in the intestine. It is known that not only IL-10 but also TGF-β has an important role in intestinal tolerance and suppression of colitis [1] , [28] , [29] . However, Tgfb1 −/− mice as well as Stat3 −/− mice with SCID or Rag -deficient backgrounds do not develop colitis [4] , [5] , [6] , [30] . We also confirmed that Il10 −/− Rag2 −/− mice do not develop colitis during our observation period (2 to 4 months after birth, Supplementary Fig. S2 ). Although Il10 −/− Rag2 −/− mice may still develop colitis with age, it is clear that IL-10 is dispensable for maintenance of intestinal tolerance in young adult lymphopenic mice. Thus, it appears that effector T cells are required for the development of colitis induced by TGF-β or IL-10/STAT3 deficiency. In contrast, Socs1 −/− mice developed colitis, especially, on a Rag2 −/− background, and their colitis was suppressed by a transfer of IL-10-producing Tregs. Therefore, the mechanism underlying the colitis induced by SOCS1 deficiency is apparently different from those mechanisms underlying the colitis induced by IL-10 and TGF-β deficiency. The situation of Socs1 −/− mice was somewhat similar to that of T-bet −/− mice [31] . T-bet −/− mice also develop colitis only on a Rag2 −/− background. However, there are also many differences between these two genotypes. In T-bet −/− Rag2 −/− mice, the dysregulation of cytokine production was confined only to TNFα, but in Socs1 −/− Rag2 −/− mice, many inflammatory cytokines were upregulated. Rectal prolapse was frequently observed in T-bet −/− Rag2 −/− mice, but was not observed at all in Socs1 −/− Rag2 −/− mice. The colitis spread from colitic T-bet −/− Rag2 −/− mice to healthy T-bet +/+ Rag2 −/− mice, but not from Socs1 −/− Rag2 −/− mice to Socs1 +/+ Rag2 −/− mice. Because the forms of colitis observed in these two mice are so different, we speculate that T-bet and SOCS1 differentially regulate the intestinal immune response. We have shown that STAT1 is antagonistic towards the PGE2/cAMP pathway. In addition, STAT6-activating cytokines IL-4 and IL-13 partly counteracted the immunosuppressive effect of cAMP in Socs1 −/− BMDCs ( Fig. 6 ). However, the molecular mechanisms of PGE2/cAMP-mediated immunosuppression and the antagonisms by STATs remain to be clarified. Recently, we reported that the transcription factor c-Fos is involved in the mechanism of cAMP-mediated immunosuppression in macrophages [19] . Another group has recently reported that A kinase-anchoring protein 95 (AKAP95), which interacts with p105 (nuclear factor-κB1), is responsible for cAMP-mediated suppression [30] . Further study is necessary to clarify the mechanisms of suppression and the antagonisms by STATs, the balance between which is regulated by SOCS1. Recent genome-wide association studies demonstrated a significant association of single-nucleotide polymorphisms within the proximity of the PTGER4 gene region, which regulate PTGER4 expression, with Crohn's disease [32] . Polymorphisms in the STAT3 gene and JAK2 promoter region also associate with IBD [33] , [34] , [35] , [36] . These studies suggest that alterations in the strength of PGE2 and JAK/STAT signalling can modulate susceptibility to IBD. Our study presented here also supports this idea, although we should be very careful in translating these results from animal studies to human disease. We have focused on the role of SOCS1 in the control of intestinal inflammation in this study. The dysregulation of cytokine signallings due to the lack of SOCS1 lead to colitis. Lack of SOCS3, another important negative feedback regulator of cytokine signallings, on the other hand, rendered macrophages and dendritic cells hyporesponsive to various Toll-like receptor stimuli because of the hyperactivation of STAT3 (refs 37 , 38 ), and the macropahge/neutrophil-specific Socs3 -conditional knockout mice were rather resistant to DSS-induced colitis [37] . Interestingly, STAT3-hyperactivated innate immune cells are anti-inflammatory in general, whereas STAT3-hyperactivated T cells, including the T cells devoid of Socs3 , are more prone to produce IL-17 (ref. 39 ), and thus mediate inflammation in certain conditions. Studies to clarify the cell type-specific roles of SOCS1 and SOCS3 and their relevance in various inflammatory settings in vivo are being conducted. Mice Socs1 −/− mice and Socs1 -KOTg mice with a C57BL/6J background had been established previously [12] . Il23a −/− mice have been described previously [40] . Rag2 −/− mice, Il10 −/− mice and Ifng −/− mice, all with a C57BL/6J background, were obtained from The Jackson Laboratory. Several lines of double knockout and triple knockout mice were generated by intercrossing. All mice were housed in an SPF animal facility at Kyushu University. All experiments using these mice were approved by and performed according to the guidelines of the animal ethics committee of Kyushu University, Fukuoka, Japan. Flow cytometry and cell sorting Cells were stained with the indicated fluorescein-conjugated Abs at concentrations of 1:200 to 1:1000, and were analysed on a FACSCalibur or FACSAria (Becton Dickinson) flow cytometer. All Abs and kits used were purchased from eBioscience. For the isolation of Tregs, CD4 + T cells were negatively selected using MACS (Miltenyi Biotec), and CD4 + CD25 high 7-AAD − cells were further purified using FACSAria. The sorted cells, which were used as Tregs, were >95% CD4 + CD25 high , and ∼ 90% of the isolated CD4 + CD25 high cells expressed Foxp3. Oral indomethacin administration Rag2 +/+ and Rag2 −/− mice were continuously fed with 40 μg ml −1 (corresponding to ∼ 10 mg kg −1 per day) of the non-selective COX inhibitor indomethacin (Nacalai Tesque) in drinking water for 8 to 10 days. To dissolve the indomethacin completely in water, 0.04% dimethyl sulfoxide and 0.2 mM NaOH were also added. The indomethacin solution was replaced every 48 h. Antibiotic treatment and PTGER4 agonist administration To remove the intestinal commensal bacteria, imipenem (50 mg kg −1 per day; Banyu Pharmaceutical) and vancomycin (50 mg kg −1 per day; Sigma-Aldrich) were continuously administered in drinking water. Imipenem + vancomycin at this dosage has been reported to effectively reduce both the aerobic and anaerobic bacteria residing in the colon of mice [41] . A PTGER4 agonist, ONO-AE1-329 (a generous gift from Ono Pharmaceutical), was injected subcutaneously twice a day at a dosage of 4 μg kg −1 body weight during the entire period of indomethacin administration. Histopathological examination The severity of each colitis case was determined according to the criteria shown in Table 1 . In preparation for immunohistochemical examination, frozen cryostat sections were fixed in acetone, blocked with mouse serum and incubated with the fluorescein-conjugated monoclonal Abs (1:100). The slides were examined through a fluorescence digital microscope (Keyence). Table 1 Histological scoring system for chronic colitis. Full size table Preparations of CMEs To extract whole molecules of the substances contained in the colonic mucosa, 0.2 g wet weight of the mucosal and submucosal layers removed from the colons were resuspended in RPMI 1640, frozen at −20°C and then thawed at 4°C. This freezing and thawing cycle was repeated three times. After the third thawing, samples were centrifuged, and the supernatants were filtered through a 0.22-μm filter. The liquid thus obtained was used as CME. For the comparison of PGE2 levels among tissues, several organs were collected from WT mice shortly after the euthanasia, embedded in ice-cold PBS containing 100 μM indomethacin and frozen and thawed twice. Indomethacin was included in the buffer to minimize the de novo production of PGE2 during the experimental procedure. After filtration through a 0.22-μm filter, the concentrations of proteins in the supernatants were measured and adjusted to 1 mg ml −1 . PGE2 levels of the supernatants were determined using ELISA kit (Cayman Chemical). Biochemical analysis of bone BMDCs Granulocyte-macrophage colony stimulating factor-induced BMDCs were stimulated with LPS (10 ng ml −1 , Escherichia coli serotype 055:B5, Sigma-Aldrich) in the absence or presence of the combinations of cytokines and reagents indicated in the figure legends. The levels of IL-12p70 and TNFα produced were measured with an ELISA kit (eBioscience). 8-Bromoadenosine 3,5′-cyclic monophosphate sodium salt (8-Br-cAMP) was purchased from Sigma-Aldrich. PGE2 was purchased from Nacalai Tesque. Recombinant murine cytokines were purchased from Peprotech. Anti-IL-10 Ab was purchased from eBioscience. A PTGER4 antagonist, ONO-AE3-208 is a gift from Ono Pharmaceutical. Western blot analysis Anti-tyrosine-phosphorylated STAT1 and anti-serine-phosphorylated IκBα monoclonal Abs were purchased from Cell Signaling Technology. Anti-STAT1, anti-IκBα, anti-c-Fos and anti-p65 Ab were purchased from Santa Cruz Biotechnology. Anti-actin Ab was purchased from Sigma-Aldrich. Reverse transcription PCR analysis Total RNAs from cell and tissue specimens were reverse transcribed and analysed by semi-quantitative PCR or quantitative real-time PCR. Quantitative real-time PCR was performed using the Power-SYBR Green Real-time PCR Master Mix (Applied Biosystems) and the ABI 7000 Sequence Detector System (Applied Biosystems). The comparative threshold cycle (Ct) method was used to calculate the relative expression levels of the target genes compared with the internal control ( Hprt1 ). The primer sequences are shown in Supplementary Table S1 . Statistical analysis Statistical analysis was performed using Student's t -test. A P -value <0.05 was considered to indicate statistical significance. How to cite this article: Chinen, T. et al . Prostaglandin E2 and SOCS1 have a role in intestinal immune tolerance. Nat. Commun. 2:190 doi: 10.1038/ncomms1181 (2011).